Phenotypic characterization of missense polymerase-δ mutations using an inducible protein-replacement system Next-generation sequencing has revolutionized the search for disease-causing genetic alterations. Unfortunately, the task of distinguishing the handful of causative mutations from rare variants remains daunting. We now describe an assay that permits the analysis of all types of mutations in any gene of choice through the generation of stable human cell lines, in which the endogenous protein has been inducibly replaced with its genetic variant. Here we studied the phenotype of variants of the essential replicative polymerase-δ carrying missense mutations in its active site, similar to those recently identified in familial colon cancer patients. We show that expression of the mutants but not the wild-type protein endows the engineered cells with a mutator phenotype and that the mutations affect the fidelity and/or the exonuclease activity of the isolated enzyme in vitro . This proof-of-principle study demonstrates the general applicability of this experimental approach in the study of genotype–phenotype correlations. Hereditary non-polyposis colon cancer or Lynch syndrome accounts for ~4% of all colorectal cancers and segregates predominantly with mutations in the MMR genes MSH2 and MLH1 (ref. 1 ). Cell lines isolated from MMR-deficient tumours have a mutator phenotype and display microsatellite instability [2] . Puzzlingly, nearly two decades ago, analysis of eight microsatellite instability-positive colon cancer cell lines that were not mutated in the MSH2 or MLH1 loci failed to reveal mutations in the remaining MMR genes known at that time , PMS1 and PMS2 . Instead, a heterozygous mutation was found in the POLD1 gene [3] , which encodes the catalytic subunit of polymerase-δ (pol-δ), the enzyme primarily responsible for lagging strand synthesis [4] and DNA repair [5] . The link of this mutation to malignancy has not been tested because the cell line concerned (DLD1/HCT15) was soon thereafter shown to harbour a mutation in the newly discovered MMR gene MSH6 (ref. 6 ). However, heterozygous mutations in POLD1 have since been shown to predispose to cancer in mouse models [7] and the most recent identification of mutations in pol-δ and pol-ε (the leading strand polymerase) in familial colon cancer patients [8] implies that these genetic alterations are likely to be causative. Owing to the essential nature of replicative polymerases, the disease-causing mutations will be predominantly amino-acid substitutions rather than frameshifts or stop codons, and this will make it difficult to distinguish them from rare variants or polymorphisms. Similarly, nearly 1/3 of MMR gene mutations in Lynch syndrome families carry missense mutations [1] . Although several attempts were made to design reporter systems capable of distinguishing causative mutations from rare variants [9] , the assays are complex and their readouts can be unreliable. We therefore set out to develop a facile system capable of characterizing the phenotypic consequences of genetic alterations affecting genes such as POLD1 and MLH1 . To this end, we decided to make use of interfering RNA (RNAi) and inducible gene expression. The development of RNAi technology has revolutionized mammalian genetics. Transient transfection of cells with synthetic small interfering RNAs (siRNAs) mediates short-term knockdown of the targeted mRNAs and thus allows analysis of phenotypes associated with gene inactivations by mutations ranging from premature stop codons through out-of-frame insertions and deletions to epigenetic silencing. The study of medium-to-long-term effects is best achieved with short hairpin RNA (shRNA), which offers several important advantages over siRNA [10] . It is expressed from plasmid or viral vectors, which makes it possible to establish stable cell lines that express the shRNA either constitutively or inducibly. shRNA is also substantially cheaper than siRNA. An important shortcoming of RNAi technology are off-target effects [11] ; however, specificity can be demonstrated by rescue of the observed phenotype through expression of an RNAi-resistant mRNA [12] , [13] . Originally designed as a control experiment to check the specificity of RNAis, this approach has been extended to deploy RNAi-resistant mRNAs to express protein variants. Thus, by downregulating the endogenous mRNA by RNAi, the phenotype of a given mutation could be studied in the absence of the wild-type (WT) protein. This above approach has often met with success; yet, it has a number of limitations. It requires several lengthy and laborious selection steps, particularly where long-term effects are being studied. Most importantly, single, stable clones expressing both the shRNA and the RNAi-resistant mRNA have to be isolated to ensure that the cells express both the variant and the WT control. This raises the possibility that the observed phenotypic differences are caused by clonal differences rather than by the different functions of the two proteins. We now describe a method that overcomes these shortcomings. We generated a plasmid vector we refer to as all-in-one (pAIO), which can express both the shRNA- and the RNAi-resistant mRNA encoding the polypeptide of interest from tetracycline-inducible promoters. When stably transfected into cell lines expressing the tetracycline repressor, expression of the variant protein and the concomitant knockdown of the endogenous polypeptide can be achieved simply by the addition of Doxycycline (Dox). In this way, the effect of the variant protein on the phenotype of the cells can be reversibly studied in an identical genetic background. We demonstrate the feasibility of the approach by analysing the phenotype of cells in which the catalytic subunit of DNA polymerase-δ was replaced with variants carrying mutations affecting the fidelity of the enzyme and/or its exonuclease proofreading function, similar to those recently identified in familial colon cancer patients. We show that protein replacement resulted in decreased replication efficiency and fidelity in vivo , as well as in measurable defects in exonuclease activity in vitro, as anticipated. The concept of inducible protein replacement Given the essential nature of pol-δ, we argued that its knockdown with shRNA, followed by stable transfection with the variant cDNA, would not be feasible. We therefore set out to design a system that would permit a gradual replacement of the endogenous enzyme with the exogenous variant. To achieve this goal, we modified the tetracycline-inducible shRNA vector pSUPERIOR (OligoEngine Inc.) by inserting into it an additional tetracycline operator-binding site, a CMV enhancer/promoter and a multiple cloning site. Once this vector is charged with the desired shRNA and cDNA inserts, and stably integrated into genomic DNA of a cell line expressing the tetracycline repressor (Invitrogen), addition of Dox to the medium induces the expression of both the shRNA and the mRNA encoding the protein of interest. By targeting the shRNA specifically to the endogenous mRNA, the endogenous protein will be replaced by the exogenous variant once the former had been naturally degraded (most proteins have half-lives in the range of 1–4 days). All-in-one vectors encoding pol-δ WT and mutant variants We decided to test the functionality of our ‘protein-replacement’ system by substituting the catalytic subunit of pol-δ with several mutant variants. Pol-δ is a heterotetramer; its p66, p50 and p12 subunits contribute to replication fidelity; however, p125, encoded by the POLD1 gene, plays the key role in replication. It not only carries the polymerase active site that controls the selection of the incoming nucleotide with an error rate of ~1 per 10 5 ; it also contains the proofreading exonuclease activity, which removes nucleotides misincorporated at the 3′ termini of nascent DNA and thus improves polymerase error rate by a further two orders of magnitude. Biosynthetic errors that escape the proofreading function are addressed by the MMR system, which improves replication fidelity by a further three orders of magnitude. We therefore wondered whether substitution of the endogenous high-fidelity p125 subunit with variants carrying missense mutations in the polymerase active site or in the proofreading function previously demonstrated to exhibit a hypermutator phenotype in vitro and in vivo [14] would give rise to a cell line with a clear mutator phenotype even in cells with a fully functional MMR system. We created four different pAIO vectors ( Fig. 1a ) encoding 3 × FLAG-tagged p125, either WT, error-prone (EP), proofreading-deficient (PD) or the double mutant (DM). The EP variant, L606G, was shown to alter the selectivity of the polymerase for the incoming dNTPs [15] . The PD variant carries a D402A amino-acid substitution that is equivalent to the D400A mutation used previously to inactivate the proofreading function of murine pol-δ [16] . Both mutations are highly conserved among all B family polymerases and have been shown in yeast and in mouse models to have a mutator phenotype [17] , [18] . The DM variant harbours both the D402A and the L606G mutations. In addition, silent mutations were introduced into the p125 cDNA at the shRNA target sequence, which render the exogenous p125 mRNA resistant to the shRNA ( Fig. 1a,b ). In order to ensure that the phenotypes resulting from expression of the p125 variants were not linked to off-target effects of the shRNA or caused by the silent mutations in the cDNA, we also constructed a vector encoding the WT p125 cDNA containing the same silent mutations as the variants. 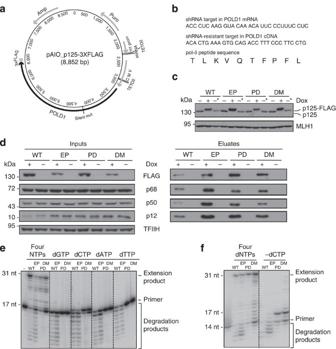Figure 1: Expression and biochemical characterization of the polymerase-δ variants. (a) Schematic representation of the pAIO vector. Open reading frames encoding the antibiotic resistance markers (Amp, Puro), the pol-δ cDNA (POLD1), the positions of the double tetracycline operator (TET02)-binding sites in the H1 and the CMV promoter sequences, as well as the position of the 3 × FLAG tag and the site of the silent mutations (see alsob) are indicated. (b) Target of the shRNA in endogenous pol-δ mRNA (top row) and silent mutations introduced into the pol-δ cDNA that render the exogenous mRNA resistant to the same shRNA (middle row). The pol-δ peptide sequence remains unaltered by the mutations (bottom row). (c) Western blot of extracts of stable clones expressing either the endogenous pol-δ (−Dox lanes) or the FLAG-tagged variant (lanes+Dox). Note that the presence of the 3 × FLAG tag retards the migration of the polypeptides through the denaturing polyacrylamide gels. When the Dox-treated cells were replated in Dox-free medium, the endogenous pol-δ polypeptide was re-expressed (−*Dox lanes). MLH1 was used as the loading control. (d) Induction of exogenous pol-δ expression by Dox does not alter the expression levels of the p68, p50 and p12 pol-δ subunits (left panel). TFIIH was used as the loading control. The 3 × FLAG-tagged p125 pol-δ subunit associates with the remaining subunits of the enzyme in pull-down experiments (right panel). (e) Pol-δ isolated from the variant cell clones by affinity purification on a FLAG column is enzymatically active in a primer extension assay, using a 31-mer template and a 17-mer primer. In this ‘standing start’ assay, all four variants incorporate only dCMP opposite the G at position 18 of the template. The PD and DM variants lack proofreading exonuclease activity, as witnessed by the lack of 17-mer degradation products in reactions containing these polypeptides. (f) The variants are active in a ‘running start’ assay, in which a 14-mer primer was annealed with a 31-mer template and incubated with the polymerases in the presence of all four dNTPs (left panel). The right panel shows the results of the same assay in which only dATP, dGTP and dTTP were provided. Figure 1: Expression and biochemical characterization of the polymerase-δ variants. ( a ) Schematic representation of the pAIO vector. Open reading frames encoding the antibiotic resistance markers (Amp, Puro), the pol-δ cDNA (POLD1), the positions of the double tetracycline operator (TET02)-binding sites in the H1 and the CMV promoter sequences, as well as the position of the 3 × FLAG tag and the site of the silent mutations (see also b ) are indicated. ( b ) Target of the shRNA in endogenous pol-δ mRNA (top row) and silent mutations introduced into the pol-δ cDNA that render the exogenous mRNA resistant to the same shRNA (middle row). The pol-δ peptide sequence remains unaltered by the mutations (bottom row). ( c ) Western blot of extracts of stable clones expressing either the endogenous pol-δ (−Dox lanes) or the FLAG-tagged variant (lanes+Dox). Note that the presence of the 3 × FLAG tag retards the migration of the polypeptides through the denaturing polyacrylamide gels. When the Dox-treated cells were replated in Dox-free medium, the endogenous pol-δ polypeptide was re-expressed (−*Dox lanes). MLH1 was used as the loading control. ( d ) Induction of exogenous pol-δ expression by Dox does not alter the expression levels of the p68, p50 and p12 pol-δ subunits (left panel). TFIIH was used as the loading control. The 3 × FLAG-tagged p125 pol-δ subunit associates with the remaining subunits of the enzyme in pull-down experiments (right panel). ( e ) Pol-δ isolated from the variant cell clones by affinity purification on a FLAG column is enzymatically active in a primer extension assay, using a 31-mer template and a 17-mer primer. In this ‘standing start’ assay, all four variants incorporate only dCMP opposite the G at position 18 of the template. The PD and DM variants lack proofreading exonuclease activity, as witnessed by the lack of 17-mer degradation products in reactions containing these polypeptides. ( f ) The variants are active in a ‘running start’ assay, in which a 14-mer primer was annealed with a 31-mer template and incubated with the polymerases in the presence of all four dNTPs (left panel). The right panel shows the results of the same assay in which only dATP, dGTP and dTTP were provided. Full size image Cell lines inducibly expressing pol-δ variants The above vectors were transfected into A2780-TRex cells, an ovarian cancer cell line that had been generated in our laboratory by transfecting the MMR-proficient A2780-MLH1 (ref. 9 ) parental cell line with a vector stably expressing the tetracycline repressor (Invitrogen). As shown in Fig. 1c , we obtained cell lines that, upon induction with Dox (+), expressed the different FLAG-tagged p125 variants and that contained substantially reduced levels of the endogenous p125. This phenotype was reversible; we cultured the cells in Dox for 4 days, followed by further 4 days without it. After removal of the drug, exogenous p125 ceased to be expressed in all four cell lines, while endogenous p125 reappeared ( Fig. 1c , lanes –*). Importantly, the replacement of p125 with the FLAG-tagged variants affected neither the levels of MLH1 ( Fig. 1c ), protein required for MMR, nor did p125-FLAG expression affect the levels of the other subunits of the pol-δ heterotetramer ( Fig. 1d , left panel). Biochemical characterization of pol-δ variants That the FLAG-tagged p125 interacted with the other pol-δ subunits was shown in pull-down experiments using an anti-FLAG antibody and total extracts of the Dox-induced cell lines. As shown in Fig. 1d (right panel), all four subunits were detected in the immunoprecipitates from Dox-treated cells. In order to test whether these FLAG-tagged pol-δ complexes were functional, we isolated them by affinity chromatography using beads derivatized with an anti-FLAG antibody. The complexes were then eluted with the FLAG peptide and used in primer extension assays using a 17-mer primer annealed to a 31-mer template. In the presence of all four dNTPs, the full-length (31-mer) extension products were observed ( Fig. 1e ), but only in eluates obtained from extracts of Dox-treated cells. As anticipated, the reaction was stimulated by the addition of proliferating-cell nuclear antigen (PCNA), the processivity factor of replicative polymerases ( Supplementary Fig. 1a ). We also observed exonucleolytic degradation of the primer but only in eluates containing the WT and EP pol-δ variants ( Fig. 1e ). This indicated that the D402A mutation in the PD and DM variants indeed inactivated the exonuclease activity. Moreover, the result also showed that the eluates were not appreciably contaminated with endogenous polymerases or nucleases. In these so-called ‘standing start’ primer extensions, all four polymerase variants were unable to insert a non-complementary nucleotide at the end of the primer. Thus, when only one of the four dNTPs was provided, dCMP was the sole nucleotide incorporated opposite the template dG at the +1 position ( Fig. 1e ). This changed in the ‘running start’ assay, where a 14-mer primer was used, and where the nucleotide pool was limited to three dNTPs. In this assay, the polymerase had the correct nucleotides for the first two elongation steps, but the correct nucleotide for the third step, dCTP, was omitted. As shown in Fig. 1f , the WT and EP variants failed to extend the primer efficiently. Moreover, the EP variant caused substantial degradation of the 14-mer, most likely because it frequently misinserted wrong nucleotides in place of the missing dCMP, which activated the proofreading exonuclease. The PD and DM variants, which lack the exonuclease activity, efficiently extended the primer to a 17-mer. Moreover, the DM variant generated also some full-length extension product. This finding agrees with published data [19] and can be explained by the fact that the L606G mutation increases the size of the active site of p125, which helps to accommodate non-complementary nucleotides and extend from them but only in the absence of proofreading. Taken together, our characterization of the FLAG-tagged pol-δ variants isolated by affinity chromatography from human cells showed that all four enzymes were active and that their biochemical properties reflected those described for recombinant variants produced in heterologous systems. These results demonstrate that our protein replacement approach is applicable also to the study of phenotype–genotype correlations of essential protein–gene combinations in human cells. Increased mutation rates in cells expressing pol-δ variants In Escherichia coli , the mutD5 mutation in the dnaQ gene encoding the proofreading exonuclease of the DNA pol III holoenzyme exhibited a potent mutator phenotype that saturated the capacity of the MMR pathway [20] . We wondered whether expression of the mutator p125 variants compromised MMR in human cells. In the first instance, we tested the MMR capacity of extracts generated from the Dox-induced cells. As shown in Supplementary Fig. 1b , all extracts were MMR-proficient; this finding confirmed that the MMR system was intact in these cells and further confirmed that the exogenous pol-δ variants were able to carry out repair synthesis, the penultimate step of the MMR process [21] . In yeast [22] , [23] and mice [7] , [16] , expression of pol-δ mutants analogous to those studied here brought about an increase in spontaneous mutation rates and, in the mouse, predisposition to cancer. These results suggested that the MMR system was unable to deal with the increased load of mutations, similarly to what was observed in E. coli [20] . In order to learn whether this was the case also in human cells, we measured the spontaneous mutation rates of our cell lines at the hypoxanthine–guanine phosphoribosyl transferase ( HPRT ) locus. As shown in Table 1 , replacement of endogenous pol-δ with the tagged WT variant in A2780-TRex cells did not affect the mutation rates when compared with the parental cell line [9] . In contrast, the spontaneous mutation rates of the EP and PD clones were elevated 8- and 13-fold, respectively, and that of the DM clone was 17-fold higher. The latter increase is close to that measured in the MMR-deficient A2780 derivative [9] , which suggests that the low fidelity of the DM variant saturated the MMR capacity of the cells. Table 1 Number of cultures ( n ), final number of cells at time of selection, fraction of cultures with no mutants ( P 0 ) and mutation rates ( μ ) at the HPRT gene in the indicated cell lines. Full size table Replication stress in cells expressing pol-δ variants In order to learn whether the increase in mutation rates affected progression of the cells through the S phase, we pulse-labelled the newly synthesized DNA with 5-ethynyl-2′-deoxyuridine (EdU). As shown in Fig. 2a , EdU incorporation was similar in all four clones grown without Dox. Upon addition of Dox, EdU incorporation in the EP and DM clones was substantially diminished, whereas that of the WT and PD clones was largely unaffected. This indicated that the error-prone polymerase slows down the progression of the replication forks, as observed previously [19] . We therefore wondered whether this might activate an S phase checkpoint. We pulse-labelled the cells with EdU and performed immunofluorescence experiments using a γ-H2AX antibody, which is widely used to mark sites of DNA damage, particularly double-stranded breaks (DSBs). We observed an increased number of γ-H2AX foci in the S phase (EdU-positive) cells expressing the active-site mutants but not the WT or the PD variants ( Fig. 2b ). The γ-H2AX foci co-localized with those of RPA ( Supplementary Fig. 2a ) and 53BP1 ( Supplementary Fig. 2b ), accepted markers of DSB processing. These findings were substantiated by western blotting analysis, where extracts of the EP and DM clones displayed strong phosphorylation of KAP1, a target of the ATM kinase that helps decondense damaged chromatin and aids in the recruitment of repair factors such a 53BP1to sites of DSBs ( Fig. 2c ). Interestingly, we detected no appreciable phosphorylation of CHK1, a downstream target of ATR kinase, which is recruited and activated by ATR-interacting protein that binds to RPA-coated single-stranded DNA regions at arrested replication forks [24] . This was unexpected because hydroxyurea treatment, which blocks replication by depleting nucleotide pools through inhibiting ribonucleotide reductase, readily activates both ATR and ATM, and gives rise to γ-H2AX-, RPA- and 53BP1 foci [25] . Our current finding thus indicates that the molecular mechanisms of delayed S phase progression induced by nucleotide depletion or by the error-prone polymerases differ. 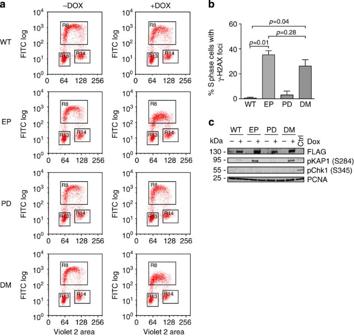Figure 2: Cell cycle progression and checkpoint activation in clones inducibly expressing pol-δ variants. (a) Two-dimensional FACS analysis of cell populations stained with 4,6-diamidino-2-phenylindole (abscissa) and EdU (ordinate). The untreated cell (−Dox) clones progressed through the cell cycle similarly. Upon induction of the pol-δ variant expression (+Dox), S phase progression of the EP and DM clones was retarded. (b) Progression through the S phase gave rise to spontaneous foci of γ-H2AX in the EP and DM clones that largely co-localized with foci of RPA and 53BP1 (see alsoSupplementary Fig. 2). The graph represents EdU-positive cells displaying γ-H2AX foci. More than 50 nuclei were counted in two independent experiments and the data are represented as mean±s.e.m.Pvalues were calculated using unpaired two-tailedt-test. (c) Expression of the EP and DM polypeptides was also accompanied by the activation of the ATM kinase, as indicated by phosphorylation of its downstream target KAP1. The replication-dependent kinase ATR was not activated in these cells, as witnessed by the lack of phosphorylation of its downstream target Chk1. Ctrl, extracts of UV-treated cells, positive control of ATR activation. Figure 2: Cell cycle progression and checkpoint activation in clones inducibly expressing pol-δ variants. ( a ) Two-dimensional FACS analysis of cell populations stained with 4,6-diamidino-2-phenylindole (abscissa) and EdU (ordinate). The untreated cell (−Dox) clones progressed through the cell cycle similarly. Upon induction of the pol-δ variant expression (+Dox), S phase progression of the EP and DM clones was retarded. ( b ) Progression through the S phase gave rise to spontaneous foci of γ-H2AX in the EP and DM clones that largely co-localized with foci of RPA and 53BP1 (see also Supplementary Fig. 2 ). The graph represents EdU-positive cells displaying γ-H2AX foci. More than 50 nuclei were counted in two independent experiments and the data are represented as mean±s.e.m. P values were calculated using unpaired two-tailed t -test. ( c ) Expression of the EP and DM polypeptides was also accompanied by the activation of the ATM kinase, as indicated by phosphorylation of its downstream target KAP1. The replication-dependent kinase ATR was not activated in these cells, as witnessed by the lack of phosphorylation of its downstream target Chk1. Ctrl, extracts of UV-treated cells, positive control of ATR activation. Full size image Stress response of cells expressing pol-δ variants The differences in replication stress apparent from the slower progression of the EP and DM clones through the S phase relative to cells expressing the WT and PD pol-δ variants failed to affect cell viability. We therefore wanted to learn how the four cell clones respond to exogenous DNA damage. To this end, we challenged them with ultraviolet radiation (UV), or with the methylating agents methyl-methanesulfonate (MMS) and N -methyl- N′ -nitro- N -nitrosoguanidine (MNNG). Cells maintained without Dox were treated similarly and served as controls. As shown in Fig. 3a , the clones were similarly sensitive to UV. In contrast, the EP and DM clones displayed an increased sensitivity to MMS ( Fig. 3b ), as observed also for S. cerevisiae strains carrying analogous mutations [7] . The exonuclease-deficient PD mutant was not more sensitive than the WT clone, which could have been anticipated based on the fact that MMS produces primarily N 7 -methylguanine and N 3 -methyladenine in DNA, which form Watson–Crick base pairs and are thus unlikely to be detected by the proofreading function. However, both methylated bases are prone to spontaneous or enzymatic cleavage of the glycosidic bond, which gives rise to highly toxic abasic sites in the DNA. Bypass of these sites generally requires specialized polymerases such as Rev1 and pol-ζ (ref. 26 ). Unsuccessful attempts of the EP and DM polymerases to bypass these lesions might be the underlying reason for the greater cytotoxicity of MMS in cells expressing these variants. 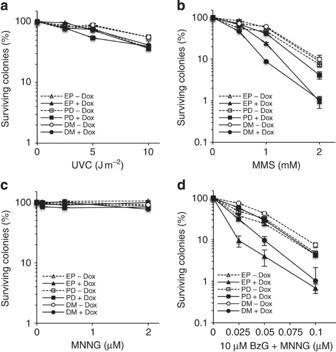Figure 3: Differential sensitivity of pol-δ variant-expressing clones to DNA-damaging agents. Clonogenic cell viability assays documenting the toxicity of increasing doses of UV radiation (a), MMS (b) or MNNG (without (c) or with (d) pretreatment with BzG). All cell clones grown in the absence of doxycycline (−Dox) responded similarly to these agents. Upon induction of expression of the pol-δ variants (+Dox), the EP and DM clones became hypersensitive to MMS and MNNG, but not to UV. Each data point represents an average±s.d. of treatment conditions carried out in triplicates. Figure 3: Differential sensitivity of pol-δ variant-expressing clones to DNA-damaging agents. Clonogenic cell viability assays documenting the toxicity of increasing doses of UV radiation ( a ), MMS ( b ) or MNNG (without ( c ) or with ( d ) pretreatment with BzG). All cell clones grown in the absence of doxycycline (−Dox) responded similarly to these agents. Upon induction of expression of the pol-δ variants (+Dox), the EP and DM clones became hypersensitive to MMS and MNNG, but not to UV. Each data point represents an average±s.d. of treatment conditions carried out in triplicates. Full size image In contrast to MMS, MNNG is toxic to cells at much lower concentrations, because of its ability to generate, in addition to N 7 -methylguanine and N 3 -methyladenine, also O 6 -methylguanine (MeG) in DNA. These modifications are efficiently repaired by methylguanine methyltransferase; however, when the enzyme is absent or inhibited by O 6 -benzylguanine (BzG), MeGs persist in the DNA, where they trigger MMR-mediated cycles of futile repair that lead to cell death. This hypothesis is supported by a wealth of evidence showing that MMR-deficient cells are highly resistant to killing by MNNG [21] . Correspondingly, in the absence of BzG pretreatment, all clones were insensitive to MNNG up to 2 μM concentration ( Fig. 3c ). This demonstrates that N 7 -methylguanine and N 3 -methyladenine levels were too low to be toxic (MMS is also not toxic at this concentration), and that MeGs were efficiently repaired by methylguanine methyltransferase. In contrast, pretreatment with BzG sensitized the cells to much lower MNNG concentrations ( Fig. 3d ), which indicated that the observed toxicity was linked to the persistence of MeG in the DNA and that MMR was functional in these cells. The EP and DM clones were particularly sensitive, which suggested that the EP polymerase variants generated substrates that gave rise to more cytotoxicity when addressed by MMR. The experimental ‘protein-replacement’ system described above has been developed with the intention to facilitate genotype–phenotype studies, particularly those involving missense mutations. By selecting pol-δ for our proof-of-principle study, we were able to demonstrate that this technology can be used to ‘replace’ even an essential protein. Moreover, because the phenotypes of similar or analogous mutations in pol-δ have been tested in other model organisms [7] , [16] , [17] , we were able to verify the results obtained in our system. In addition, we show that our experimental set-up permits not only the phenotypic characterization of the stable cell lines but also the analysis of the biochemical properties of the protein variants and their interactomes. Importantly, this system is fully isogenic, inasmuch as the study is carried out in a single cell line either treated or not with doxycyclin, rather than in different clones. The phenotypic switch is also reversible; withdrawal of Dox results in the substitution of the variant with the endogenous WT protein and the cell will revert to its original phenotype, unless the expression of the variant protein generated irreversible changes in the cells, such as mutations in the genomic DNA generated by mutant pol-δ in the present study. The reversibility of the phenotypic switch, as well as the ease of studying any type of mutation, represents an advantage of our system over the most recent technologies of genome editing such as ZFN, TALEN or CRISPR (see ref. 27 for review). The latter approaches readily generate targeted genomic deletions, which cause full gene inactivation by non-homologous end-joining rather than a knockdown achieved by shRNA, but the introduction of specific mutations via homologous recombination is substantially less efficient, and requires expensive and time-consuming screening for correct clones. Moreover, the system is not reversible, and rescue experiments require transfection of the cells with plasmid or bacmid vectors followed by clonal selection [12] , [13] , which could introduce artifacts. Our system controls for off-target effects of the shRNA by including a control that expresses the tagged WT variant in the presence of the shRNA. In addition, our system can be further simplified by targeting the shRNA to sequences in the 3′-untranslated regions of the respective mRNAs. Unfortunately, this option was not available to us because of the lack of a suitable RNAi target in the 3′-untranslated region of p125 mRNA. We therefore had to target our shRNA to the coding sequence of p125, which required site-directed mutagenesis. In addition to generating a novel tool for the study of genotype–phenotype correlations, our results also led to an interesting finding. The general dogma of DNA replication posits that the fidelity of this key process of DNA metabolism is controlled by three principal factors: accuracy of the DNA polymerase, its proofreading ability and MMR. The question that puzzled us concerned the substrate specificity of the proofreading function and its interplay with MMR in vivo. Does the proofreading function address all errors made by the polymerase, or only those mispairs that cannot be extended from, as suggested by in vitro studies [28] ? In addition, does MMR address all mispairs generated by the polymerase and not eliminated by its proofreading function? That the mutation frequency of the PD mutants was more than 10-fold elevated ( Table 1 ) suggested that the MMR system failed to repair all errors of the polymerase. The system was not saturated because the PD mutant was sensitized to MNNG treatment, which requires functional MMR. We therefore propose that the proofreading function addresses primarily non-Watson–Crick base pairs at the end of the primer strand that the polymerase cannot easily extend from, whereas the MMR system addresses the remaining errors. Thus, rather than functioning in series, with MMR acting downstream from proofreading, the two functions appear to work in parallel. Finally, our data also suggest that MMR can be saturated, as demonstrated by the finding that the mutator phenotype of the DM clones ( Table 1 ) was similar to that of MMR-deficient clones derived from the same cell line [9] . Cell lines MMR-proficient human ovarian cancer A2780 cells (clone-MLH1-1) were obtained from Margherita Bignami (Rome). Cells were grown in Dulbecco’s Modified Eagle’s Medium (DMEM, GIBCO-BRL) supplemented with 5% Tet-approved fetal bovine serum (FBS-superior, Biochrom AG), 100 U ml −1 penicillin, 100 μg ml −1 of streptomycin (GIBCO-BRL), 1 μg ml −1 puromycin and 10 μg ml −1 blasticidin and 100 μg ml −1 G418. All the cell lines were cultured at 37 °C and 5% CO 2 . Where required, Dox (10 ng ml −1 , Sigma) was added to the medium at least 4 days before analysis. Vector construction The pAIO vectors carrying inserts encoding the pol-δ p125 subunit variants with 3 × FLAG tags at the C termini ( Fig. 1a ) were constructed by standard cloning procedures. The full vector sequence is available upon request. The silent mutations introduced into the p125 sequence that render it siRNA-resistant are shown in Fig. 1b . Cell transfections MMR-proficient human ovarian cancer A2780 cells (clone-MLH1-1) were transfected with pcDNA6/TR plasmid (Invitrogen) encoding the tet-repressor. Stable clones expressing high levels of the repressor were selected with 10 μg ml −1 blasticidin. These were then transfected with the AIO vectors encoding the Dox-inducible pol-δ variants. Stable clones were selected with puromycin (1 μg ml −1 ). Cell extracts and western blot analyses Cells were lysed in Laemmli sample buffer (4% SDS, 20% glycerol, 120 mM Tris-HCl, pH 8.0) by heating for 5 min at 95 °C. Before loading, the samples were sonicated and briefly centrifuged. The protein samples were separated by SDS–PAGE and blotted on polyvinylidene difluoride membranes. The blots were blocked with 5% non-fat powdered milk in 0.1% TBS-T (0.1% Tween-20 in TBS) for 30 min and incubated with appropriately diluted primary antibodies in 0.1% TBS-T overnight at 4 °C. Immunoblotting was carried out using the following antibodies at the indicated dilutions: p125 (Abcam, 1:1,000), p50 (a kind gift of Ulrich Hübscher, 1:1,000), p68 (Abnova, 1:1,000), p12 (Abnova, 1:200), KAP1 pS284 (A300-274A; Bethyl Laboratories Inc., 1:1,000), CHK1 pS345 (no. 2348; Cell Signaling Technology, 1:1,000), PCNA (PC10, Santa Cruz Biotechnology, 1:1,000) and MLH1 (Oncogene, 1:1,000). The membranes were incubated with the appropriate secondary horseradish peroxidase-conjugated antibodies for 1 h at room temperature. Immunoprecipitations These were carried out using Triton cell lysates obtained from cells expressing the different variants of p125. Briefly, 20 15-cm dishes were maintained for 4 days in 10 ng ml −1 Dox. Cells were harvested and lysed in Triton lysis buffer (50 mM Tris-HCl, pH 7.5, 150 mM NaCl, 1% Triton-X-100, 1 mM phenylmethyl sulphonyl fluoride, 1 × complete inhibitory mixture EDTA free (Roche), 1 mM sodium orthovanadate, 1 mM sodium fluoride, 1 mM EDTA). Lysates (20 mg) were rotated with FLAG-M2 magnetic beads in 1 ml Triton extraction buffer for 3 h at 4 °C. The beads were washed four times with wash buffer (50 mM Tris-HCl, pH 7.5, 150 mM NaCl and 1% Triton-X-100). The proteins were eluted with 100 μl elution buffer (25 mM HEPES, pH 7.8, 50 mM KCl, 0.1 mM EDTA, 10% sucrose, 2 mM dithiothreitol (DTT)) containing 300 ng μl −1 of FLAG peptide. Eluates (5 μl) were resolved on SDS–PAGE as described above. Primer extension assays The running start assays were carried out using a 32 P-labelled 14-mer primer 5 ′- CTCAAGCTTCCCAA-3 ′ annealed to the 31-mer template oligonucleotide 5′-CCAGACGTCTGTC G ACCTTGGGAAGCTTGAG-3′. The standing start assays were carried out using a 32 P 5′-labelled 17-mer primer 5′-CTCAAGCTTCCCAAGGT-3′ annealed to the same template. The position of the G where the misincorporation efficiency was tested is indicated in bold and underlined. The primer extension reactions contained 10 fmol of the annealed substrate in 50 mM bis-Tris (pH 6.5), 12.5 mM HEPES-KOH (pH 7.5), 25 mM KCl, 10 mM MgCl 2 , 5% sucrose, 0.025 mg ml −1 of bovine serum albumin, 1.5 mM DTT, 0.05 mM EDTA and, where indicated, 25 μM dNTPs and 0.1 μM PCNA in a total volume of 5 μl. The reactions were initiated by the addition of 5 μl of the p125-variant eluates. They were incubated for 10 min at 37 °C, quenched with 1 μl stop solution (1% SDS, 140 mM EDTA, 1 mg ml −1 of protK) and stopped by heating at 55 °C for 15 min. The samples were then precipitated overnight with ethanol at −20 °C, dried, the pellets were dissolved in loading buffer (95% formamide, 20 mm EDTA), heated at 95 °C for 5 min and loaded on a 20% denaturing polyacrylamide gel. The product bands were quantified using PhosphorImager analysis. Mutation rate analysis at the HPRT gene This was performed as described previously [29] . Briefly, the cells were plated at low density (100 per dish) and grown in complete medium to a density of ~0.5 × 10 6 per dish. The entire cultures (50–60 independent sets) were then transferred to a medium supplemented with 6-thioguanine (5 μg ml −1 ; Sigma). The mutation rates were calculated as μ = MC −1 ln2, where C is the number of cells at selection time and M is −ln ( P 0 ), where P 0 is the proportion of cultures with no mutants. Immunofluorescence microscopy A2780-Trex cells expressing the p125-variant constructs were cultured in 10 ng ml −1 of Dox for 4 days. The cells were then pulsed with 10 μM EdU for 15 min, after which the EdU-positive cells were detected using a Click-IT EdU kit (Invitrogen) and co-stained with an anti-γH2AX antibody (rabbit polyclonal, Cell Signaling Technology). The number of cells exhibiting γH2AX foci in EdU-positive cells were quantified. For γH2AX and RPA co-localization studies, cells maintained in Dox for 4 days were first pre-extracted for 5 min on ice (25 mM Hepes, pH 7.4, 50 mM NaCl, 1 mM EDTA, 3 mM MgCl 2 , 300 mM sucrose and 0.5% Triton-X-100) and then fixed with 4% formaldehyde (w/v) in PBS for 12 min. The coverslips were washed with PBS and then co-immunostained with primary antibodies against γH2AX (rabbit polyclonal, Cell Signaling Technology) in combination with an antibody against RPA2 (mouse monoclonal, Lab Vision). For γH2AX and 53BP1 co-localization studies, the procedure was as described above, except that the cells were fixed with 4% formaldehyde (w/v) in PBS and permeabilized with Triton before treatment with the primary antibodies. After incubation with the primary antibody, the slides were probed with the appropriate secondary antibodies (FITC, TR, 1:750, 1:250) for 1 h at room temperature. DNA was stained with 4′,6-diamidino-2-phenylindole. Slides were viewed and analysed using an Olympus IX81 microscope. FACS analysis For EdU incorporation experiments, cells were maintained in 10 μg ml −1 of Dox or not for 4 days. On the day of incubation, 10 μM EdU was added for 30 min. The cells were trypsinized and 0.5 × 10 6 cells were collected and processed for FACS using a Click-IT EdU kit (Invitrogen). Clonogenic survival assays A total of 500–1,000 cells were seeded in triplicates. After 18 h, the cells were treated with different DNA-damaging agents as indicated in the respective figure legends. After 10 days, the surviving cells were fixed and stained with 0.5% crystal violet in 20% ethanol, and colonies containing more than 50 cells were counted. The number of colonies at each drug dose was expressed as a percentage of the untreated control. How to cite this article: Ghodgaonkar, M. M. et al. Phenotypic characterization of missense polymerase-δ mutations using an inducible protein-replacement system. Nat. Commun. 5:4990 doi: 10.1038/ncomms5990 (2014).